Bright and fast multicoloured voltage reporters via electrochromic FRET Genetically encoded fluorescent reporters of membrane potential promise to reveal aspects of neural function not detectable by other means. We present a palette of multicoloured brightly fluorescent genetically encoded voltage indicators with sensitivities from 8–13% Δ F / F per 100 mV, and half-maximal response times from 4–7 ms. A fluorescent protein is fused to an archaerhodopsin-derived voltage sensor. Voltage-induced shifts in the absorption spectrum of the rhodopsin lead to voltage-dependent nonradiative quenching of the appended fluorescent protein. Through a library screen, we identify linkers and fluorescent protein combinations that report neuronal action potentials in cultured rat hippocampal neurons with a single-trial signal-to-noise ratio from 7 to 9 in a 1 kHz imaging bandwidth at modest illumination intensity. The freedom to choose a voltage indicator from an array of colours facilitates multicolour voltage imaging, as well as combination with other optical reporters and optogenetic actuators. Membrane voltage acts on all transmembrane proteins: the membrane electric field pulls on charged residues, shifting the free energy landscape for charge-displacing conformational transitions [1] . This bioelectric modulation is most famously observed in voltage-gated ion channels in neurons and cardiomyocytes, but voltage also affects the activity of G protein-coupled receptors and some transmembrane enzymes [2] . Membrane voltage is dynamically regulated in bacteria [3] , fungi [4] , plants [5] and many cell types and subcellular organelles in the human body, and is dysregulated in states of neuronal, cardiac and metabolic diseases. Thus, there is a need for fast, sensitive, bright and spectrally tunable reporters of membrane voltage. Recent progress in genetically encoded voltage indicators (GEVIs) has led to several classes of proteins, which robustly report action potentials (APs) in cultured neurons. The first GEVIs were based on fusion of fluorescent proteins to transmembrane voltage-sensing domains [6] . In some of these, voltage modulates the brightness of a single fluorescent moiety [7] , [8] , [9] , [10] , while in others, voltage modulates the efficiency of Förster resonance energy transfer (FRET) between a pair of fluorescent moieties [11] , [12] . In our measurements of green fluorescent protein (GFP)-based GEVIs, described below, the most sensitive was ArcLight [8] (Δ F / F =−32% per 100 mV), but this reporter had half-maximal response times at room temperature of 90 ms (depolarizing step) and 104 ms (hyperpolarizing step). We measured the recently introduced ASAP1 (ref. 9 ) reporter to have a sensitivity of Δ F / F =−29% per 100 mV, and a half-maximal response of 2 ms at room temperature. These numbers differ modestly from the original reports, likely due to differences in gene expression protocols and choices of optical filters. A second class of GEVIs is based on microbial rhodopsin proton pumps [3] , [13] , [14] . In these, the transmembrane voltage modulates the endogenous near infrared fluorescence of the retinal chromophore. The most recently developed non-pumping mutants of Archaerhodopsin 3 (Arch), termed QuasArs, have voltage sensitivities between 30 and 90% per 100 mV (depending on the mutant), and half-maximal response times between 50 μs and 1.1 ms at room temperature [13] . GFP-based and rhodopsin-based GEVIs have very different spectral properties. GFP-based GEVIs are excited by blue light (470–490 nm) and emit green (500–530 nm). QuasArs are excited by red light (594–640 nm) and emit in the near infrared (peak at 715 nm). GFP-based GEVIs are 30–80-fold brighter, and thus are typically imaged with excitation at ~10 W cm −2 , while QuasArs are typically imaged at 300–800 W cm −2 (ref. 13 ). In a comparison between ArcLight and QuasAr2 in cultured rat hippocampal neurons under their respective standard imaging conditions, QuasAr2 reported single APs with 4.7-fold higher signal-to-noise ratio (SNR) and was 15-fold more photostable [13] . In organotypic mouse hippocampal slice culture, QuasAr2 reported single APs with 4.5-fold higher SNR than ArcLight [13] . Nonetheless, the low brightness of Arch-based GEVIs present a challenge for widespread use. The availability of GEVIs spanning the visible spectrum is important when combining GEVIs with other optical reporters or optogenetic actuators. Having GEVIs of colours between GFP and Arch would facilitate multiplex voltage imaging, for example, to distinguish activity of excitatory and inhibitory neurons in intact tissue. Furthermore, GEVIs spectrally distinct from GFP could be paired with other GFP-based reporters such as GCaMP (Ca 2+ ) (ref. 15 ), iGluSnFR (glutamate) [16] , Perceval (ATP) [17] , Clomeleon (Cl − ) (ref. 18 ) or Pyronic (pyruvate) [19] , or with other blue-excited optogenetic actuators. Thus, there is strong motivation to develop a broad palette of GEVI colours. We sought to combine the speed and sensitivity of Arch-based GEVIs with the brightness and spectral range of conventional fluorescent proteins. Traditionally, FRET is used to measure the physical distance between a donor and acceptor. However, we and others have also used FRET to measure changes in the absorption spectrum of a protein via its influence on nonradiative quenching of an attached fluorescent moiety [20] , [21] , [22] . Here we use voltage-induced changes in the absorption spectrum of an Arch mutant to alter the degree of nonradiative quenching of a closely fused fluorescent protein. We call this mechanism electrochromic FRET (eFRET). We demonstrate fast and sensitive voltage sensing in fusions between QuasAr2 and a broad palette of fluorescent proteins: enhanced GFP (EGFP), yellow FP (Citrine), mOrange2, mRuby2. These probes have sensitivities from 8–13% Δ F / F per 100 mV, and half-maximal response times from 4–7 ms, which allows detection of APs in cultured rat hippocampal neurons with a single-trial SNR from 7 to 9 in a 1 kHz imaging bandwidth at modest illumination intensity. A recent paper applied a similar strategy to make voltage sensors based on fusion of fluorescent proteins to a mutant of the Leptosphaeria maculans rhodopsin (Mac) [23] . While other GEVIs offer superior SNR on the blue and far red ends of the spectrum, the present GEVIs fill in the visible spectrum with emission wavelengths between 530–640 nm. This spectral range facilitates multicolour voltage imaging with GEVIs, as well as combination with other optical reporters and optogenetic actuators [1] . Engineering eFRET GEVIs Our electrochromic quencher is a mutant of Arch, termed QuasAr2 ( Fig. 1 ). 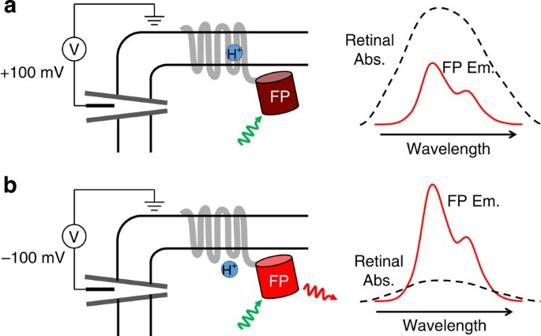Figure 1: Proposed mechanism of voltage-dependent fluorescence in eFRET GEVIs. Voltage controls the protonation, and thereby the absorption spectrum, of the Schiff base joining the retinal to the protein scaffold. (a) At a depolarizing (positive) voltage, the microbial rhodopsin has a protonated retinal Schiff base, which absorbs strongly with a peak near 600 nm. The retinal absorption quenches the fluorescence of the appended fluorescent protein (FP). (b) At hyperpolarizing (negative) voltages, the fluorescence is not quenched. Spectra shown are cartoons to illustrate mechanism. The direct retinal fluorescence of QuasAr2 showed voltage sensitivity of 90% Δ F / F per 100 mV and a bi-exponential step response with time constants of 1.2 ms (68%) and 11.8 ms (32%) ( Table 1 ) at room temperature [13] . It has not been feasible to measure directly the voltage-dependent absorption spectra of Arch or its mutants on account of the small quantity of protein found in the plasma membrane of a single cell. However, a mechanistic study of Arch showed that membrane voltage modulated fluorescence via a voltage-dependent shift in the acid-base equilibrium of the retinal Schiff base [24] . Positive membrane voltage favoured the protonated (and fluorescent) state. One can thus mimic the voltage-induced absorption changes by changing the pH in a solution of solubilized protein. At neutral pH, QuasAr2 had a broad absorption band peaked at 587 nm. At higher pH, this band dropped and a band at 411 nm appeared, corresponding to the deprotonated Schiff base ( Supplementary Fig. 1 ). Figure 1: Proposed mechanism of voltage-dependent fluorescence in eFRET GEVIs. Voltage controls the protonation, and thereby the absorption spectrum, of the Schiff base joining the retinal to the protein scaffold. ( a ) At a depolarizing (positive) voltage, the microbial rhodopsin has a protonated retinal Schiff base, which absorbs strongly with a peak near 600 nm. The retinal absorption quenches the fluorescence of the appended fluorescent protein (FP). ( b ) At hyperpolarizing (negative) voltages, the fluorescence is not quenched. Spectra shown are cartoons to illustrate mechanism. Full size image Table 1 Voltage-sensing properties of GEVIs. Full size table Based on these spectra, we reasoned that QuasAr2 might mediate voltage-dependent quenching of an appended fluorescent protein. The emission spectrum of mOrange2 (ref. 25 ) has a high degree of overlap with the absorption spectrum of Arch, so we started with this fluorophore. To enable efficient FRET, it is critical to optimize the length of the linker, as rate of FRET is proportional to the reciprocal sixth power of the distance between the donor and acceptor chromophores. We examined the crystal structures of Arch-2 (a QuasAr2 homologue) (PDB ID 2EI4) (ref. 26 ) and mOrange (an mOrange2 homologue) (PDB ID 2H5O) [27] , and found that the last 15 carboxy-terminal residues of Arch-2 and 15 amino-terminal residues of mOrange are largely unstructured ( Fig. 2a ). We reasoned that those unstructured residues could be removed without disrupting the function of either protein. We created a series of linker libraries by systematically truncating these resectable regions ( Fig. 2b and Methods) and randomizing two residues at the junction. 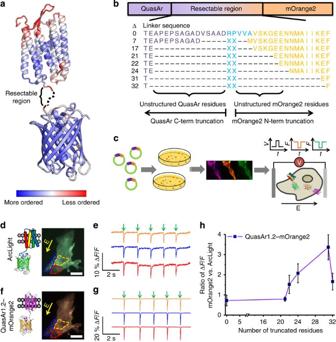Figure 2: Directed evolution of an eFRET GEVI. (a) A model of QuasAr–mOrange2 constructs, represented by the crystal structures of Arch-2 (PDB ID 2EI4)ref.26and mOrange (PDB ID 2H5O)27. The color scale represents the degree of order in the crystal structure, as reported by the B-factor. Less-ordered regions are presumed more dispensable. (b) Design of linker truncation libraries. QuasAr1.2, the best available variant at the time of the screen, was used as the electrochromic quencher. (c) Hierarchical screen of truncated linker libraries for eFRET GEVIs. Constructs were first screened inE. colifor mOrange2 brightness and then screened for membrane trafficking in HEK cells. Voltage sensitivity was then tested via field stimulation in HeLa cells co-expressing the eFRET GEVI, ArcLight (as an internal control), and Kir2.1 (to lower the resting voltage to −60 mV42). (d) ArcLight fluorescence of three HeLa cells. Yellow arrow indicates direction of the applied electric field. Scale bar, 25 μm. (e) Fluorescence intensity traces of the three regions shown ind. (f) mOrange2 fluorescence from the same cells shown ind. (g) Response of mOrange2 fluorescence during stimulation as ine. Fluorescence traces show single-trial measurement of cells imaged at 100 frames per second. (h) Effect of linker length on voltage sensitivity in QuasAr1.2–mOrange2. For each linker length the most sensitive eFRET GEVI construct was compared with ArcLight measured in the same cells. Error bars represent s.d. overn=15–20 cells in the ratio ΔF/F. Figure 2: Directed evolution of an eFRET GEVI. ( a ) A model of QuasAr–mOrange2 constructs, represented by the crystal structures of Arch-2 (PDB ID 2EI4)ref. 26 and mOrange (PDB ID 2H5O) [27] . The color scale represents the degree of order in the crystal structure, as reported by the B-factor. Less-ordered regions are presumed more dispensable. ( b ) Design of linker truncation libraries. QuasAr1.2, the best available variant at the time of the screen, was used as the electrochromic quencher. ( c ) Hierarchical screen of truncated linker libraries for eFRET GEVIs. Constructs were first screened in E. coli for mOrange2 brightness and then screened for membrane trafficking in HEK cells. Voltage sensitivity was then tested via field stimulation in HeLa cells co-expressing the eFRET GEVI, ArcLight (as an internal control), and Kir2.1 (to lower the resting voltage to −60 mV [42] ). ( d ) ArcLight fluorescence of three HeLa cells. Yellow arrow indicates direction of the applied electric field. Scale bar, 25 μm. ( e ) Fluorescence intensity traces of the three regions shown in d . ( f ) mOrange2 fluorescence from the same cells shown in d . ( g ) Response of mOrange2 fluorescence during stimulation as in e . Fluorescence traces show single-trial measurement of cells imaged at 100 frames per second. ( h ) Effect of linker length on voltage sensitivity in QuasAr1.2–mOrange2. For each linker length the most sensitive eFRET GEVI construct was compared with ArcLight measured in the same cells. Error bars represent s.d. over n =15–20 cells in the ratio Δ F / F . Full size image We then developed a hierarchical screening strategy to identify variants with optimal mOrange2 brightness, membrane trafficking and voltage response ( Fig. 2c and Methods). We used a customized vector, termed pcDuEx1.0, for gene expression in both prokaryotic and eukaryotic cells. This vector circumvents the laborious cloning typically required to switch between a primary screen in bacteria and a secondary screen in mammalian cells (Methods). Colonies of Escherichia coli were transformed with linker libraries in pcDuEx1.0. The colonies with the brightest mOrange2 fluorescence were picked for secondary screening in mammalian cells. For the mammalian cell-based screen, a green GEVI, ArcLight Q239 (ref. 7 ), was used as an internal reference for both membrane trafficking and voltage response ( Fig. 2c–g and Methods). The sensitivity of eFRET variants generally increased as the linker was shortened. The most truncated variants (Δ31 and Δ32 libraries) had excellent voltage sensitivity, but substantially decreased brightness of mOrange2, likely due either to poor folding or to high basal quenching by the rhodopsin. In libraries with more than 20 residues truncated, the screen favoured combinations of Arg, Leu, Ala and Gly for the linker. The variant from the Δ24 library with linker sequence ‘Leu-Arg’ gave the best overall performance and was used henceforth. We added a trafficking sequence (TS) and endoplasmic reticulum export motif (ER2) to improve trafficking to the plasma membrane [28] , although trafficking remained imperfect. QuasAr2 absorbs strongly from 500–640 nm, so we reasoned that eFRET might work for fluorescent proteins with a range of emission wavelengths. We created a palette of eFRET constructs by replacing mOrange2 with: ECFP [29] , EGFP [29] , Citrine [30] , mRuby2 (ref. 12 ) and mKate2 (ref. 31 ). The emission spectra of these proteins all overlapped to some degree with the absorption spectrum of QuasAr2 ( Fig. 3 ). Spectral properties of these fluorophores are given in Supplementary Table 1 . 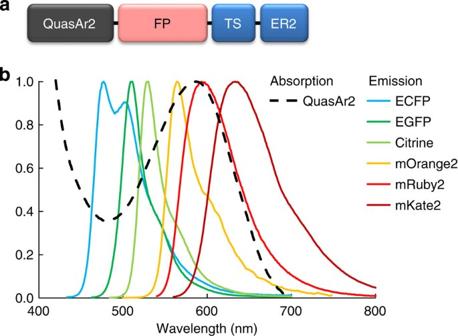Figure 3: Spectral overlap of fluorescent proteins with QuasAr2 absorption. (a) eFRET GEVI domain structure. (b) Overlay of the emission spectra of the fluorescent protein donors with the absorption spectrum of the QuasAr2 electrochromic quencher. Figure 3: Spectral overlap of fluorescent proteins with QuasAr2 absorption. ( a ) eFRET GEVI domain structure. ( b ) Overlay of the emission spectra of the fluorescent protein donors with the absorption spectrum of the QuasAr2 electrochromic quencher. Full size image To test the hypothesized eFRET mechanism, we compared the fluorescence quantum yield of Citrine in the eFRET fusion and in a membrane-targeted construct lacking the QuasAr2 quencher, both expressed in HEK cells. We used two-photon fluorescence excitation and time-correlated single-photon counting to determine the electronic excited state lifetime (Methods). The native Citrine protein had a lifetime of τ bare =3.47 ns, while the eFRET construct had a lifetime of τ F RET =2.83 ns ( Supplementary Fig. 2 ). This difference in lifetime confirms that an additional nonradiative decay pathway exists in the eFRET construct compared to the bare Citrine protein, which we ascribe to FRET from Citrine to retinal. The FRET efficiency is given by E FRET =1− τ FRET / τ bare , from which E FRET =0.18. Maximum voltage sensitivity occurs at E FRET =0.5, implying that further optimization of the position and orientation of the FP may improve quenching efficiency and thereby voltage sensitivity. Voltage responses in HEK cells We characterized the eFRET GEVIs in HEK cells, imaged at 23 °C. All eFRET GEVIs trafficked efficiently to the plasma membrane ( Fig. 4a ) and exhibited bright fluorescence when excited at 3 W cm −2 with appropriate excitation and emission wavelengths ( Supplementary Table 1 ). Membrane voltage was controlled via whole-cell voltage clamp. Fluorescence traces were extracted from images of cells either by manually defining a region of interest (ROI) comprising the cell body, or by using an automated pixel-weighting algorithm [14] . Both approaches gave similar results. Fluorescence responses were normalized to fluorescence at a holding potential of −70 mV (after background subtraction) and are quoted as Δ F / F . Voltage sensitivity was calculated as [ F (30 mV)− F (−70 mV)]/ F (−70 mV). While rhodopsins require retinal as a cofactor, we found that the culture medium contained sufficient retinal that voltage sensitivity was not enhanced by addition of exogenous retinal ( Supplementary Fig. 3 ). 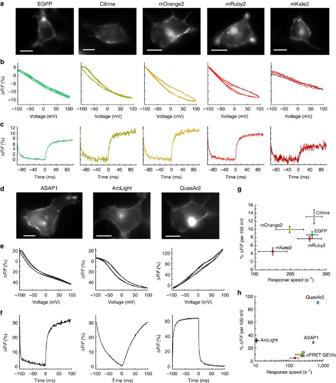Figure 4: Voltage sensing with GEVIs in HEK293 cells. Voltage response of eFRET GEVI reporters are shown in (a–c) and voltage responses of comparison GEVIs are shown in (d–f). (a,d) Fluorescence images of HEK cells expressing GEVI reporters. Scale bars, 10 μm. (b,e) Fluorescence as a function of membrane voltage, normalized to fluorescence atV=−70 mV. Many eFRET-based GEVIs showed a small amount of hysteresis. Each trace is a single trial with 100 ms exposures. (c,f) Fluorescence response to a step in membrane voltage from −70 mV to +30 mV. Each trace is averaged over 20–30 trials with 1 ms exposures. All data were acquired with laser illumination (3 W cm−2for eFRET, ASAP1 and ArcLight GEVIs, 200 W cm−2for QuasAr2). No temporal filtering was applied. Fluorescence traces were corrected for photobleaching. (g) Quantification of eFRET GEVI sensitivity and speed. Voltage sensitivity of eFRET GEVIs approximately corresponds to the degree of spectral overlap between the emission of the GEVI and the absorption of QuasAr2. (h) eFRET GEVI sensitivity and speed in the context of other GEVIs. Response speed was defined as the inverse of the time to reach 50% of steady-state response to a voltage step from −70 mV to +30 mV. Data in (g) and (h) represents an average ofn=6–9 cells for each construct. Error bars represent s.e.m. Figure 4: Voltage sensing with GEVIs in HEK293 cells. Voltage response of eFRET GEVI reporters are shown in ( a – c ) and voltage responses of comparison GEVIs are shown in ( d – f ). ( a , d ) Fluorescence images of HEK cells expressing GEVI reporters. Scale bars, 10 μm. ( b , e ) Fluorescence as a function of membrane voltage, normalized to fluorescence at V =−70 mV. Many eFRET-based GEVIs showed a small amount of hysteresis. Each trace is a single trial with 100 ms exposures. ( c , f ) Fluorescence response to a step in membrane voltage from −70 mV to +30 mV. Each trace is averaged over 20–30 trials with 1 ms exposures. All data were acquired with laser illumination (3 W cm −2 for eFRET, ASAP1 and ArcLight GEVIs, 200 W cm −2 for QuasAr2). No temporal filtering was applied. Fluorescence traces were corrected for photobleaching. ( g ) Quantification of eFRET GEVI sensitivity and speed. Voltage sensitivity of eFRET GEVIs approximately corresponds to the degree of spectral overlap between the emission of the GEVI and the absorption of QuasAr2. ( h ) eFRET GEVI sensitivity and speed in the context of other GEVIs. Response speed was defined as the inverse of the time to reach 50% of steady-state response to a voltage step from −70 mV to +30 mV. Data in ( g ) and ( h ) represents an average of n =6–9 cells for each construct. Error bars represent s.e.m. Full size image Fluorescence of all eFRET GEVIs showed approximately linear dependence on applied voltage ( Fig. 4b ). The most sensitive construct was the Citrine fusion with Δ F / F =−13.1±1.8% per 100 mV ( n =6 cells, all statistics are mean±s.e.m.). The EGFP, mOrange2 and mRuby2 constructs showed sensitivities between 7.7 and 10.0% per 100 mV ( Table 1 ). The bluest and reddest constructs, containing ECFP and mKate2, exhibited poor voltage sensitivity, which we attribute to poor spectral overlap with QuasAr2 absorption. The negative slope of dF/dV was consistent with greater spectral overlap of mOrange2 emission and QuasAr2 absorption at depolarizing voltages. Fast fluorescence response to a change in voltage is essential for detecting neuronal APs. We applied a square wave of voltage (−70 mV to +30 mV, 5 Hz) and recorded the fluorescence at a frame rate of 1,000 frames per s ( Fig. 4c ). Fluorescence responses were approximately fit by a sum of two exponentials, with a dominant fast and a smaller slow time constant. The fastest construct was the mRuby2 GEVI, with τ fast =3.6±0.3 ms (65%) and τ slow =20±2 ms (35%) for depolarizing membrane potential step ( n =8 cells). The GFP, Citrine and mOrange2 had half-response times between 3.9 and 7.6 ms ( Table 1 ). Response times were similar on rising and falling edges. Response amplitudes to a 5 ms step from −70 to +30 mV are given in Supplementary Table 2 . We made side-by-side comparisons of the performance of the eFRET GEVIs with two GFP-based GEVIs, ArcLight Q239 (ref. 7 ), and ASAP1 (ref. 9 ), and to direct fluorescence of QuasAr2 ( Fig. 4d–f ). Cell culture, gene expression, electrophysiology, imaging and analysis protocols were identical across constructs (except for changes in illumination wavelength and intensity as noted). ArcLight showed voltage sensitivity of −31.6±3.5% ΔF/F per 100 mV ( n =7 cells, Fig. 4e ), consistent with previous reports. The step response of ArcLight followed a bi-exponential decay with time constants of 28±8 ms (39%) and 271±6 ms (61%) (for a depolarizing voltage step from −70 mV to +30 mV) and a bi-exponential fluorescence rise with time constants of 104±21 ms (61%) and 283±40 ms (39%) (for voltage step from +30 mV to −70 mV) ( n =7 cells, Supplementary Fig. 4 ). These numbers are slower than in the original report on ArcLight [7] , due to the difference in measurement temperature: 23 °C in our measurements versus 33–35 °C in the prior report. ASAP1 showed voltage sensitivity of 28.8±1.7% per 100 mV and depolarizing voltage step response time constants of 2.3±0.1 ms (88%) and 39±3 ms (12%) ( n =6 cells, Fig. 4e–f ; Table 1 ). The voltage response of direct retinal fluorescence of QuasAr2 was measured in the QuasAr2-mOrange eFRET GEVI. To achieve comparable levels of QuasAr2 and mOrange2 fluorescence required 70-fold greater illumination intensity for QuasAr2 (640 nm, 200 W cm −2 versus 532 nm, 3 W cm −2 ). Compared with the mOrange2 fluorescence, QuasAr2 fluorescence was more sensitive to voltage (Δ F / F =90±2% per 100 mV, n =6 cells, Fig. 4e–h ) and had a somewhat faster response time (double exponential fit yielding: τ 1 =1.2 ms, 68%, τ 2 =12 ms, 32%, Fig. 4e–h ). The discrepancy in response time between the QuasAr2 and mOrange2 may arise because, in addition to the fast fluorescence-determining transition, QuasAr2 may also undergo slower voltage-dependent transitions that change its absorption spectrum but not its fluorescence. Alternatively, subtle voltage-induced conformational shifts could change the relative position and orientation of the mOrange2 and the retinal, and thereby change the efficiency of nonradiative quenching. Characterization in neurons The Citrine, mOrange2 and mRuby2 eFRET GEVIs showed sufficient sensitivity and speed to merit testing in neurons. We expressed these via transient transfection in cultured rat hippocampal neurons. Constructs exhibited good trafficking to the plasma membrane ( Fig. 5 ). Injection of current pulses via a patch pipette (500–600 pA, 5–10 ms, 5 Hz) induced trains of APs, which induced downward fluorescence transients of 9.7±1.7% (Citrine), 9.9±1.3% (mOrange2) and 5.4±0.4% (mRuby2) ( n =7–11 cells for each, Table 1 ). Our eFRET constructs also reported spontaneous activity in cultured neurons ( Fig. 6 ). 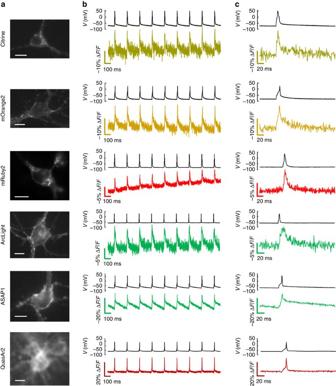Figure 5: Single-trial recording of neuronal APs with GEVIs. Each GEVI construct was expressed in primary rat hippocampal neurons under a CaMKIIα promoter. APs were induced by current injections through a patch pipette. (a) Images of neurons expressing the indicated GEVI. Scale bars, 10 μm. (b) Simultaneous patch clamp and fluorescence recordings of AP waveforms. All recordings were acquired with laser illumination (3 W cm−2for eFRET, ASAP1, and ArcLight GEVIs, 200 W cm−2for QuasAr2) at an exposure time of 1 ms. Fluorescence traces are presented without temporal filtering nor correction for photobleaching. All but the QuasAr2 recording have been inverted (hence photobleaching appears as an upward trend in the mRuby2 trace). Recordings are representative traces from 5–11 cells recorded for each construct. (c) Close-up showing single trial, unfiltered, electrically and optically recorded AP waveforms. Figure 5: Single-trial recording of neuronal APs with GEVIs. Each GEVI construct was expressed in primary rat hippocampal neurons under a CaMKIIα promoter. APs were induced by current injections through a patch pipette. ( a ) Images of neurons expressing the indicated GEVI. Scale bars, 10 μm. ( b ) Simultaneous patch clamp and fluorescence recordings of AP waveforms. All recordings were acquired with laser illumination (3 W cm −2 for eFRET, ASAP1, and ArcLight GEVIs, 200 W cm −2 for QuasAr2) at an exposure time of 1 ms. Fluorescence traces are presented without temporal filtering nor correction for photobleaching. All but the QuasAr2 recording have been inverted (hence photobleaching appears as an upward trend in the mRuby2 trace). Recordings are representative traces from 5–11 cells recorded for each construct. ( c ) Close-up showing single trial, unfiltered, electrically and optically recorded AP waveforms. 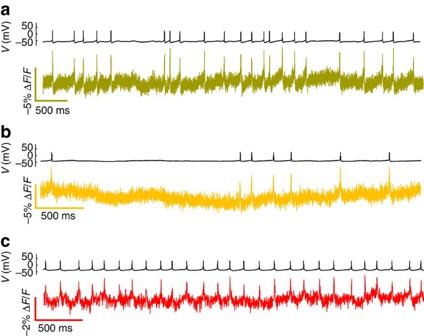Figure 6: Optical recording of spontaneous neuronal firing with eFRET GEVIs. In neurons synaptically coupled to a spontaneously active circuit, the (a) Citrine, (b) mOrange and (c) mRuby2 eFRET GEVIs clearly revealed single APs. Patch clamp voltage recordings are shown above optical recording traces. All recordings were acquired with laser illumination (3 W cm−2) at an exposure time of 2 ms. Fluorescence traces are presented without temporal filtering. The optical recordings have been corrected for photobleaching with a linear fit. Full size image Figure 6: Optical recording of spontaneous neuronal firing with eFRET GEVIs. In neurons synaptically coupled to a spontaneously active circuit, the ( a ) Citrine, ( b ) mOrange and ( c ) mRuby2 eFRET GEVIs clearly revealed single APs. Patch clamp voltage recordings are shown above optical recording traces. All recordings were acquired with laser illumination (3 W cm −2 ) at an exposure time of 2 ms. Fluorescence traces are presented without temporal filtering. The optical recordings have been corrected for photobleaching with a linear fit. Full size image Arclight also reported single-trial APs when used at 23 °C, with a downward transient of 8.2±0.7% ( n =7 cells), although this response appeared to be dominated by the response to the slow subthreshold depolarization as opposed to the fast spike. Thus, despite the greater steady-state voltage sensitivity of ArcLight than the eFRET GEVIs, the slow response of ArcLight acted as a low-pass filter on millisecond-timescale APs, decreasing the fluorescence response [7] . ASAP1 reported single-trial neuronal APs with downward fluorescence transients of 17.8±3.4% ( n =5 cells). On account of its greater sensitivity at negative voltages, ASAP1 magnified the subthreshold signal (55% of fluorescence response) relative to the AP spike (45% of fluorescence response). In a similar assay, Mac-based eFRET GEVIs were reported to resolve single APs with downward transients of 7.2% for MacQ–mOrange2 and 4.8% for MacQ-mCitrine [23] . The SNR of fluorescence detection, defined as the ratio of the peak amplitude to s.d. of fluorescence at the baseline, was 8.8±1.0 (Citrine), 9.0±1.2 (mOrange2) and 7.2±0.6 (mRuby2) (1 kHz frame rate, illumination at 3 W cm −2 , 23 °C for all eFRET GEVIs) ( n =7–11 cells for each, Table 1 ). Parallel measurements on ArcLight had a single-trial SNR of 9.2±1.5 and substantially broadened the AP waveform (1 kHz frame rate, illumination at 3 W cm −2 , 23 °C), while ASAP1 had a single-trial SNR of 13.1±2.9. Previous measurements with QuasAr2 reported a single-trial SNR for AP detection of 41 (300 W cm −2 ) and 70 (800 W cm −2 ) (ref. 13 ). With the proliferation of GEVI constructs, it can be difficult to identify the best construct for a particular experiment. Speed, sensitivity and SNR for single APs for recently reported GEVIs are summarized in Table 1 . SNR depends on both voltage sensitivity (Δ F / F ) and overall fluorescence counts ( F ). In the shot noise-limited regime, SNR for AP detection scales as , where Δ F is the change in fluorescence counts for a single AP. Baseline fluorescence counts, F , can vary considerably between experiments, depending upon illumination intensity and wavelength, protein expression level, sources of background autofluorescence, collection efficiency of the objective, choice of emission filter, quantum efficiency of the detector and selection of the ROI. The SNR values reported here provide a comparative guide for measurements under matched conditions, but will differ for measurements performed under different conditions. For multicolour voltage imaging, the choice of emission filter is critical. We used the noise scaling to estimate the SNR for each eFRET GEVI for 30 nm-wide detection bands between 510–690 nm. We then determined which eFRET GEVI gave the maximum SNR in each band ( Supplementary Fig. 5 ). This calculation suggests that the eFRET GEVIs enable detection of APs with SNR>5 for any 30 nm emission band between 510–660 nm. In the GFP spectral band, ASAP1 outperforms the eFRET GEVIs and ArcLight in terms of sensitivity, speed and SNR. In the yellow and orange emission bands, the MacQ-based eFRET GEVIs [23] are somewhat more sensitive, while the QuasAr2-based eFRET GEVIs are somewhat faster. For detection of APs in cultured neurons, both types of constructs yield similar SNR. At the far red end of the spectrum, QuasAr2 outperforms both ASAP1 and the eFRET GEVIs in terms of sensitivity, speed, SNR and photostability; but requires intense laser illumination. The excitation and emission wavelengths of a GEVI or other optical reporter influence performance when imaging in intact tissue. The excitation and emission spectra of flavins, a major contributor to brain autofluorescence, overlap strongly with those of GFP [32] , [33] . Consequently, a rule of thumb is that the signal-to-background ratio for GFP-based reporters is 10-fold lower in tissue than in cell culture. Redder reporters have significantly less background in brain tissue. Light scattering in tissue scales with wavelength λ approximately as λ −2.33 , so redder reporters can be imaged deeper [34] . Illumination at 640 nm propagates nearly 1.9-fold further into tissue than does illumination at 488 nm. While two-photon excitation of GFP-based reporters enables even greater depth penetration, this comes at the cost of requiring serial scanning, and a complex optical setup. Absolute brightness is also important when imaging in tissue, due to the need to overcome background autofluorescence and to minimize optical power dissipation in the tissue. However, in a comparison between ArcLight and QuasAr2 in rat brain slice, the far dimmer but redder QuasAr2 reported APs with 4.5-fold higher SNR than ArcLight, albeit at 24-fold higher illumination intensity [13] . Due to the complex combination of factors that determine GEVI performance in vivo , an empirical test is far preferable to extrapolations from measurements in vitro . Trafficking remains a key limitation of all GEVIs, despite adoption of trafficking motifs in most. The efficiency of trafficking to the plasma membrane often varies dramatically between preparations, between cells of the same type in vitro versus in vivo , and between different cell types from the same species. For now, an empirical approach is warranted to identify the construct best suited to a particular experiment. The varied F versus V curves for available GEVIs accentuate different aspects of cellular electrophysiology. The more linear GEVIs (eFRET and QuasArs) preserve the waveform of the underlying voltage dynamics, a useful feature for quantification of action potential waveforms. The more sigmoidal GEVIs (ASAP1 and ArcLight) emphasize voltage changes in the region of maximum slope. For ASAP1 and ArcLight this feature would emphasize subthreshold dynamics over APs in population-level recordings averaged over many cells. Due to their slightly different voltages of maximum slope, ASAP1 would show greatest sensitivity for hyperpolarizing potentials while ArcLight would show greatest sensitivity for depolarizing potentials ( Fig. 4e ). ArcLight variants have been demonstrated with maximum sensitivity over a range of voltages [7] . Several challenges remain in genetically encoded voltage imaging. Owing to uncontrolled variation in expression level, none of the GEVIs discussed here reports absolute membrane voltage. To achieve absolute accuracy requires a more complex imaging scheme, either ratiometric [35] or time-resolved [36] . Two-photon voltage imaging, which would facilitate imaging in tissue, also remains a challenge. This goal has been achieved with voltage-sensitive dyes [37] , but two-photon GEVI imaging has not yet clearly resolved single APs, although some recent work succeeded in detecting activity-evoked signals [38] . Further improvements in the eFRET GEVIs are likely to come from optimization of the rhodopsin-based quencher and from improvements in the attachment of the fluorescent protein to the rhodopsin. A rhodopsin need not show endogenous fluorescence to serve as an efficient eFRET quencher, and thus many rhodopsins that are not suitable as direct voltage indicators may still be useful for eFRET. Thousands of microbial rhodopsin genes have been identified in the wild [39] , [40] , and among these improved quenchers are likely to exist. The estimated FRET efficiency of 18% in the Citrine construct implies that increases in voltage sensitivity could be attained by improving energy transfer from the fluorescent protein to the rhodopsin. This increase in efficiency could come from greater intimacy of contact between the fluorescent protein and the rhodopsin, or from optimizing the relative orientation of the donor and acceptor fluorophores. To achieve these goals, one may insert circularly permuted fluorescent proteins into intracellular loops on the rhodopsin. With simultaneous multicolour voltage imaging, one could apply genetic targeting to record voltage simultaneously from distinct structures that might otherwise be difficult to distinguish. For instance, wide-field images that lack single-cell resolution could still distinguish population-average activity levels in intermingled excitatory and inhibitory neurons. The broad palette of eFRET GEVIs also facilitates combination with other GFP-based fluorescent reporters or a wide variety of optogenetic actuators. Molecular biology Synthetic DNA oligonucleotides were purchased from Integrated DNA Technologies. PfuUltraII polymerase (Agilent Technologies) or Phusion Polymerase (New England Biolabs) were used for high fidelity PCR amplifications in the buffer supplied by the respective manufacturer. PCR products and products of restriction digests were purified either with PCR clean up kit (Qiagen) or using preparative agarose gel electrophoresis followed by DNA isolation using the Zymoclean gel DNA recovery kit (Zymo Research). Restriction endonucleases were purchased from New England Biolabs and used according to the manufacturer’s instructions. Ligations were performed using T4 DNA ligase (Invitrogen) or Gibson Assembly (New England Biolabs). Small-scale isolation of plasmid DNA was performed by plasmid Miniprep kit (Qiagen). The cDNA sequences for all fusion constructs were confirmed by sequencing (Genewiz). Site-directed mutagenesis was performed with QuikChange kit (Agilent Technologies). Construction of linker libraries A vector for expression in prokaryotic and eukaryotic systems was constructed based on mammalian expression vector pcDNA3.1 (+). To facilitate prokaryotic expression, a customized constitutive promoter was introduced 5′-ttgctttgtgagcggataacaattataatagattca-3′ based on the phage early T5 promoter for prokaryotic transcription [41] . An E. coli ribosome binding site 5′-aggaggaa-3′ for prokaryotic translation was also introduced via QuikChange reactions. The resultant vector, designated pcDuEx1.0, exhibits moderate expression of Arch-mOrange2 fusions in E. coli cells and very similar expression levels in HeLa cells compared with its predecessor. We used pcDuEx1.0 as the vector for screening of linker libraries. We focused on mOrange2 fusions for determining optimized linker length for FRET efficiency. We chose QuasAr1.2 (Arch D95N/D106H, the best available at the time of the screen) as the Arch body. For construction of QuasAr1.2–mOrange2 Δ0, we fused QuasAr1.2 to the N terminus of mOrange2 fusion via a 5 residue linker (RPVVA) using overlap PCR. The DNA was PCR amplified with the flanking restriction sites BamHI and XbaI, followed by double digestion and ligation into pcDuEx1.0 linearized by digestion with the same two enzymes. From the template of QuasAr1.2–mOrange2 Δ0, we constructed linker libraries by systematic truncation of the connecting region between QuasAr1.2 and mOrange2 using Quikchange reactions ( Fig. 2 ). For each library, two randomized amino-acid residues (nucleotide sequence NNKNNK, where N =A, G, C, T and K =G, T) were placed between the C terminus of Arch and the N terminus of mOrange2, to generate 400 amino-acid combinations (1024 nucleotide combinations). The libraries were cloned into pcDuEx1.0 via standard procedure of restriction enzyme digestion and ligation. Hierarchical screen of linker libraries E. coli (DH10B, Invitrogen) colonies expressing the linker library exhibited varied intensities of mOrange2 fluorescence. For each library, the 24 variants with brightest mOrange2 fluorescence were picked and grown in overnight culture at 37 °C. The plasmid DNA of each variant was prepared from overnight culture using standard miniprep procedure. For each variant, the plasma membrane trafficking was examined in HEK cells (CRL-1573, ATCC) co-expressing ArcLight, which served as internal reference. The five variants with the best membrane trafficking were then expressed in HeLa cells for testing of voltage sensitivity. HeLa cells (CCL2, ATCC) were grown to 40–60% confluence on home-made 35 mm glass-bottom dishes or 24-well glass-bottom plates, and transfected with 1 μg of plasmid DNA and 2 μl Turbofect (Thermo Scientific) according to the manufacturer’s instructions. HeLa cells were transfected with plasmids encoding the QuasAr1.2–mOrange2 variant, ArcLight Q239 (Addgene: 36856) and Kir2.1 (Addgene: 32641) in equal weight ratio. Expression of Kir2.1 in HeLa cells maintained the resting potential close to −60 mV, appropriate for a neuronal voltage indicator [42] . After 3 h incubation, the media was exchanged to DMEM with 10% fetal bovine serum and the cells were incubated for an additional 24 h at 37 °C in a CO 2 incubator. Immediately before imaging, cells were washed twice with Hanks balanced salt solution and then 1 ml of 20 mM HEPES-buffered Hanks balanced salt solution was added. No retinal was added to the buffer–loading of retinal into the rhodopsin was presumed to occur from endogenous retinal. Cell imaging was performed with an inverted Eclipse Ti-E (Nikon) equipped with a Photometrics QuantEM 512SC camera and a 150 W mercury-xenon lamp (Hamamatsu). A home-made parallel platinum electrode pair with a separation distance of 0.5 cm was mounted in a custom plastic support and was placed in the imaging dish or well. The waveforms of voltage pulses were generated by a pulse generator PG 58A (Gould Advance) and amplified by an Agilent 6824A 40V/25A DC Power Supply (Hewlett Packard). The typical waveform had square wave pulses lasting 20 ms with pulse field strength ranging from 50–60 V cm −1 . The mOrange2 fluorescence was imaged at 100 Hz frame rate in 4 × 4 binning mode for 10 s using the following filter set: 545/30 nm (excitation), 620/60 nm (emission) and 565 nm (dichroic). For imaging ArcLight, the filter set was: 480/40 nm (excitation), 535/40 nm (emission) and 505 nm (dichroic). The raw fluorescence traces of both mOrange2 and ArcLight were extracted from identical regions of interest in cells expressing both constructs, and exported into a Microsoft Excel spreadsheet using the microscope software NIS-Elements Advanced Research (Nikon). Background subtraction, photobleaching corrections, calculations of average Δ F / F and calculation of SNR were performed automatically in Excel. The average Δ F / F and SNR of mOrange2 signals was compared with those of ArcLight signals from the same cells, and the ratios of Δ F / F of mOrange2 versus ArcLight were reported. At least 20 cells co-expressing mOrange2 fusion and ArcLight were analysed for each variant. The best variant with maximum mean ratio in each library was determined and sequenced. pH-dependent absorption spectrum of QuasAr2 E. coli cells transformed with a pBAD vector encoding QuasAr2 were grown in 12 ml liquid LB medium with 200 μg ml −1 ampicillin overnight. The next day, 12 ml of liquid LB medium containing 50 μM retinal, 200 μg ml −1 ampicillin and 0.2% L -arabinose was added into the culture to induce expression of QuasAr2, followed by additional incubation at 37 °C for 3.5 h. The cell pellets were collected by centrifugation, washed with Tris-buffered saline (30 mM Tris, 150 mM NaCl, pH 7.4), and lysed with a tip sonicator for 10 min. The cytoplasmic fraction was discarded after centrifugation and the coloured insoluble fraction was resuspended in a series of modified Tris-buffered saline buffers (30 mM Tris, 150 mM NaCl, adjusted to the pH value of the spectral measurement) containing 1% N -dodecyl-β- D -maltopyranoside (Affymetrix). The suspension was then centrifuged (17,000 g for 15 min, 4 °C). Absorption spectra of QuasAr2 in the supernatant in different pH were recorded on a DU-800 ultraviolet-visible spectrophotometer (Beckman). Expression vectors for HEK cells and neurons We chose lentivirus vector FCK-Arch-EGFP (Addgene: 22217) as the backbone for all eFRET constructs. This vector features a CaMKIIα promoter and a Woodchuck hepatitis virus posttranscriptional regulatory element after the 3′ end of the open reading frame. To enhance membrane trafficking of fusion proteins, we added a TS and ER export signal peptide sequence (FCYENEV), derived from the inward rectifier potassium channel Kir2.1, as previously described [28] . QuasAr2-FP fusion constructs were made by Gibson Assembly: the vector was linearized by double digestion with BamHI and BsrGI, and QuasAr2 and fluorescent protein cDNA segments were generated by PCR amplification. The linker configuration of all eFRET fusion proteins was constructed based on the optimized linker sequence found by the linker screening. In all eFRET fusion proteins, the N-terminal 2 amino acids of QuasAr2 were changed from DP to VS to facilitate expression, and the C-terminal 14 amino acids of QuasAr2 (APEPSAGADVSAAD) were replaced with a 2-amino-acid linker, Leu-Arg (based on the optimized linker sequence found in linker library Δ24), to shorten the distance between QuasAr2 and fluorescent protein. The N-terminal amino acids in the fluorescent proteins were also truncated ( Supplementary Table 3 ). The nucleotide sequences of all constructs are in the Supplementary Note 1 . Two-photon lifetime measurements to determine FRET efficiency We measured fluorescence lifetime on a home-built beam-scanning two-photon microscope with an 80 MHz, 100 fs tunable pulsed laser (SpectraPhysics Insight DeepSee). Pulse compression in the sample plane was performed through maximizing the fluorescence intensity of a bead-sample, using the motorized prism compressor built into the laser. The citrine measurements were performed at 1,040 nm excitation wavelength with a time-averaged excitation power of 30 mW, or 0.4 nJ per pulse, focused down to a ~500 nm spot with a 1.2 NA water immersion objective (Olympus UplanSapo) for a time-averaged intensity of 15 MW cm −2 ; measurements were performed for linear speeds of the scanned spot varying between 0 and 30 cm s −1 without any measurable effect on fluorescence lifetime. Excitation light and fluorescence were separated using a FF775-Di01 dichroic mirror and FF01-790/SP-25 Shortpass filter (Both Semrock); fluorescence was detected using a Hamamatsu R943-02 photomultiplier tube in photon counting mode, cooled to −20 °C. The PMT signal was amplified through an SRS PR325 amplifier and discretized with a Hamamatsu Photon counting unit C9744, before being fed into a Picoharp 300 TCSPC module (Picoquant). The setup was controlled by Labview software written in-house. Simultaneous electrophysiology and fluorescence in HEK cells HEK293t/17 cells (ATCC CRL-11268) were cultured and transfected following standard protocols. Briefly, cells were grown at 37 °C, 5% CO 2 , in DMEM supplemented with 10% fetal bovine serum and penicillin–streptomycin. Plasmids were transfected using TransIT-293 reagent (Mirus Bio LLC) following the manufacturer’s instructions. Twenty-four hours post transfection, cells were re-plated onto glass-bottom dishes (MatTek) at a density of ~10,000 cells cm −2 . Cells were assayed 40–60 h post transfection. Despite the presence of saturating retinal in the culture medium, cells were supplemented with retinal before measurement to remove a possible source of variability. Cells were supplemented with retinal by preincubating with 5 μM retinal in growth medium (diluted from 40 mM stock solution in dimethyl sulphoxide) in the incubator for 0.5–1 h immediately before imaging. All imaging and electrophysiology were performed in Tyrode’s buffer (containing 125 mM NaCl, 2.5 mM KCl, 3 mM CaCl 2 , 1 mM MgCl 2 , 10 mM HEPES, 30 mM glucose, at pH 7.3 and adjusted to 305–310 mOsm with sucrose). A gap junction blocker, 2-aminoethoxydiphenyl borate (50 μM, Sigma), was added to eliminate electrical coupling between cells. Filamented glass micropipettes (WPI) were pulled to a tip resistance of 5–10 MΩ, and filled with internal solution containing 125 mM potassium gluconate, 8 mM NaCl, 0.6 mM MgCl 2 , 0.1 mM CaCl 2 , 1 mM EGTA, 10 mM HEPES, 4 mM Mg-ATP, 0.4 mM Na-GTP (pH 7.3); adjusted to 295 mOsm with sucrose. Pipettes were positioned with a Sutter MP285 manipulator. Whole-cell, voltage and current clamp recordings were acquired using a patch clamp amplifier (A-M Systems, Model 2400), filtered at 5 kHz with the internal filter and digitized with a National Instruments PCIE-6323 acquisition board at 10 kHz. Simultaneous whole-cell patch clamp recordings and fluorescence recordings were acquired on a home-built, inverted epifluorescence microscope, described below in the section ‘Imaging Apparatus’. Neuronal culture and electrophysiology All procedures involving animals were in accordance with the National Institutes of Health Guide for the care and use of laboratory animals and were approved by the Institutional Animal Care and Use Committee at the institution at which they were carried out. Hippocampal neurons from P0 rat pups were dissected and cultured in neurobasal-based medium (NBActiv4, Brainbits) at a density of 40,000 cm −2 on glass-bottom dishes (MatTek) pre-coated with poly- D -lysine (Sigma P7205) and matrigel (BD Biosciences 356234). At 3 days in vitro (DIV), cytarabine was added to the neuronal culture medium at a final concentration of 2 μM to inhibit glial growth [43] . Neurons were transfected on DIV 7 with the eFRET plasmid using Lipofectamine 2000 transfection reagent (Life Technologies). Procedures followed manufacturer’s instructions but reduced the amount of reagent by 50–80% to avoid toxicity. Measurements were performed on primary cultures at DIV 10–20. Experiments were conducted in Tyrode’s solution containing 125 mM NaCl, 2.5 mM KCl, 3 mM CaCl 2 , 1 mM MgCl 2 , 10 mM HEPES, 30 mM glucose (pH 7.3) and adjusted to 305–310 mOsm with sucrose. Immediately before imaging, neurons were incubated with 5 μM all- trans retinal in the culture medium for 30 min and then washed with Tyrode’s solution. Experiments were performed at 23 °C under ambient atmosphere. Imaging apparatus Experiments were conducted on a home-built inverted fluorescence microscope equipped with 488 nm, 532 nm, 561 nm, 594 nm and 640 nm laser lines and a scientific CMOS camera (Hamamatsu ORCA-Flash 4.0). The power and manufacturer of laser lines are summarized in Supplementary Table 4 . Illumination from lasers were combined using dichroic mirrors, sent through an acousto-optic tunable filter (Gooch and Housego 48058-2.5-.55-5W) for intensity modulation, and then expanded and focused onto the back focal plane of a × 60 water immersion objective, numerical aperture 1.20 (Olympus UIS2 UPlanSApo × 60/1.20 W). Imaging of fluorescent proteins was performed at illumination intensities of 2–4 W cm −2 . Imaging of QuasAr2-direct fluorescence was performed at an illumination intensity of 200–400 W cm −2 . Supplementary Table 5 summarizes the laser lines, dichroic mirrors and emission filters used for fluorescence imaging. For fast data acquisition, a small field of view around the cell of interest was chosen at the centre of the camera to achieve a frame rate of 1,000 frames per second. Data analysis Data was analysed with home-made software written in MATLAB. Fluorescence intensities from raw movies were extracted using a maximum likelihood pixel-weighting algorithm described in ref. 14 . Briefly, the fluorescence at each pixel was correlated with the mean fluorescence. Pixels that showed stronger correlation to the mean were preferentially weighted. This algorithm automatically found the pixels carrying the most information, and de-emphasized background pixels. Alternatively, a ROI comprising the cell body was defined by the user, and fluorescence intensity was calculated from the unweighted mean of pixel values within the ROI. With the improved trafficking of the QuasAr2 mutants resulting from the TS and ER2 motifs, the ROI approach gave similar results as the maximum likelihood pixel-weighting algorithm. For eFRET speed analysis, the time constants for the step response were calculated by fitting a double exponential to the rising and decaying portions of the fluorescence traces. All error ranges represent s.e.m. How to cite this article : Zou, P. et al . Bright and fast multicoloured voltage reporters via electrochromic FRET. Nat. Commun. 5:4625 doi: 10.1038/ncomms5625 (2014).